Wwp2 is essential for palatogenesis mediated by the interaction between Sox9 and mediator subunit 25 Sox9 is a direct transcriptional activator of cartilage-specific extracellular matrix genes and has essential roles in chondrogenesis. Mutations in or around the SOX9 gene cause campomelic dysplasia or Pierre Robin Sequence. However, Sox9 -dependent transcriptional control in chondrogenesis remains largely unknown. Here we identify Wwp2 as a direct target of Sox9. Wwp2 interacts physically with Sox9 and is associated with Sox9 transcriptional activity via its nuclear translocation. A yeast two-hybrid screen using a cDNA library reveals that Wwp2 interacts with Med25, a component of the Mediator complex. The positive regulation of Sox9 transcriptional activity by Wwp2 is mediated by the binding between Sox9 and Med25. In zebrafish, morpholino-mediated knockdown of either wwp2 or med25 induces palatal malformation, which is comparable to that in sox9 mutants. These results provide evidence that the regulatory interaction between Sox9, Wwp2 and Med25 defines the Sox9 transcriptional mechanisms of chondrogenesis in the forming palate. The initiation of mesenchymal condensation and overt chondrogenesis depend on the transcription factor Sox9. Loss-of-function and gain-of-function analyses using mouse genetic approaches have revealed that Sox9 has an essential role in successive steps of chondrogenesis that are mediated by cell proliferation, differentiation and extracellular matrix production [1] , [2] . Haploinsufficiency of SOX9 causes campomelic dysplasia, which is a severe and often lethal skeletal dysplasia associated with sex reversal [3] , [4] . Hypomorphic intragenic mutations or position effect translocation breakpoints around the SOX9 gene cause the site- and stage-specific disruption of SOX9 transcription, resulting in Pierre Robin Sequence [5] , which is characterized by micrognathis, glossoptosis and cleft palate. Indeed, heterozygous Sox9 mutant mice died perinatally with cleft palate [6] . Previous studies have showed that Sox9 induces L-Sox5 and Sox6 transcription, and these Sox proteins coordinately regulate the expression of cartilage-specific extracellular matrix genes, including Col2a1 , Col11a2 and Aggrecan [1] , [7] , [8] , [9] . Genetic variants in these genes also cause palatal malformation [10] , [11] , [12] . These findings indicate that Sox9 transcriptional activity has a regulatory role in palatogenesis. The activity of Sox9 in chondrogenesis is controlled by several transcription factors. Recently, the thyroid hormone receptor-associated protein 230/Med12 (which is a member of the Mediator complex), the nuclear RNA-binding protein, p54 nrb the CREB-binding protein (CBP)/p300, and the Tat interactive protein-60 have been reported as modulators of Sox9 transcriptional activity [13] , [14] , [15] , [16] , [17] . However, Sox9-related genes and Sox9-dependent transcriptional regulation during chondrogenesis are not fully understood. To define the repertoire of Sox9-dependent genes that contribute to the regulation of chondrogenesis, we generated Sox9-3′ enhanced green fluorescent protein (EGFP) knock-in mice and Sox9-EGFP/EGFP null chimeras, and then performed a fluorescence-activated cell sorting (FACS)/comparative microarray gene expression analysis using EGFP-positive cells derived from limb buds of the mouse embryos. Subsequently, using in situ hybridization analysis of Sox9 in limb buds of wild-type and conditional Sox9 knockout embryos harbouring the Prx1-Cre transgene, we identified genes that may be involved in chondrogenesis. Of these candidate genes, we focused on Wwp2, a member of the neural precursor cell expressed, developmentally downregulated 4-like protein family and the HECT domain E3 ubiquitin-protein ligases [18] . Wwp2 controls the epithelial Na(+) channel [19] and the divalent metal ion transporter DMT1 [20] . In addition, recent reports have showed that Wwp2 mediates Oct4 ubiquitination and degradation in embryonic stem (ES) cells [21] . However, the expression and functions of Wwp2 in chondrogenesis remain unknown. Here we demonstrate that Wwp2 interacts physically with Sox9 and Med25, mediator of RNA polymerase II transcription subunit 25, and reveal that Med25 transmits Sox9 transcriptional activity, which is mediated by binding with Wwp2. Furthermore, morpholino-mediated knockdown of either wwp2 or med25 induced palatal malformation in zebrafish, which is comparable to that observed in zebrafish sox9 mutants. These findings provide new insights into the regulatory mechanisms of Sox9 transcriptional activity in chondrogenesis. Wwp2 is identified as a Sox9-related gene in chondrogenesis To define the repertoire of in vivo Sox9-dependent genes in chondrogenesis, we performed FACS on genetically engineered mouse embryos that selectively express EGFP in a Sox9-specific pattern, followed by whole-genome microarray expression profiling on the isolated cells. For this purpose, we generated mutant mice in which an internal ribosome entry site ( IRES ) -EGFP-pA/loxP-flanked PGK-neo-bpA cassette was inserted into the 3′-untranslated region of the Sox9 gene in exon 3 just at the 5′ end to the polyadenylation signal (Sox9-3′ EGFP knock-in mice; Fig. 1a,b ). Heterozygous and homozygous Sox9-3′ EGFP knock-in mice were viable and fertile and showed no noticeable phenotypic changes. In addition, EGFP expression was detectable in a Sox9-specific pattern during embryogenesis ( Fig. 1c ). Next, we generated Sox9-EGFP/EGFP null ES cells by insertion of IRES-EGFP-pA/loxP-flanked PGK-neo-bpA cassette into the coding regions of the Sox9 gene ( Fig. 1d–g ). Our target strategy functionally inactivated Sox9 and led to the expression of EGFP in a Sox9-specific pattern. 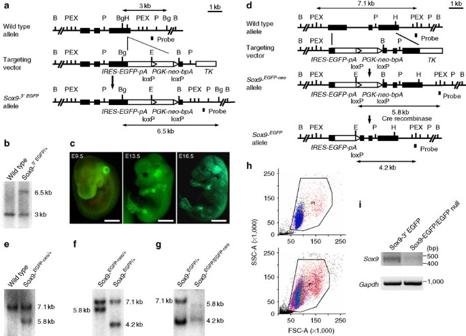Figure 1: Generation of Sox9-3′ EGFP knock-in mice and Sox9-EGFP/EGFP null chimeras. (a) The structure of the genomicSox9locus, targeting vector and targeted allele for Sox9-3′ EGFP knock-in mouse is indicated. Exons are depicted as closed boxes and intronic sequences are shown as solid lines. DNA fragments detected by Southern blot analysis are indicated by double arrows, with the restriction enzymes and the probe. TheIRES-EGFP-pA/loxP-flanked PGK-neo-bpAcassette is depicted as open boxes. B,BamHI; P,Pst1; E,EcoRI; X,XbaI; Bg,BglII; H,HpaI. (b) Southern blot analysis of genomic DNA. Genomic DNA isolated from ES cell clones was digested withBglII and was then hybridized with the 3′ probe. The wild-type and mutant alleles were detected as 3 kb and 6.5 kb fragments, respectively. (c) EGFP expression in E9.5, E13.5 and E16.5 Sox9-3′ EGFP knock-in embryos. EGFP expression was detectable in a Sox9-specific pattern during embryogenesis. Scale bars, 500 μm (E9.5); 2 mm (E13.5) and 3 mm (E16.5). (d) The structure of the genomicSox9locus, targeting vector and targeted allele for Sox9-EGFP/EGFP null chimera is indicated. DNA fragments detected by Southern blot analysis are indicated by double arrows. (e) Southern blot analysis of genomic DNA. Genomic DNA isolated from ES cell clones was digested withEcoRI and was then hybridized with the 3′ probe. Wild-type and mutant alleles were detected as 7.1 kb and 5.8 kb fragments, respectively. (f) Southern blot analysis of the neo-deleted Sox9 EGFP clones after Cre recombination. The neo-deleted Sox9 EGFP allele was detected as a 4.2 kb fragment. (g) Southern blot analysis of the neo-deleted Sox9 EGFP/EGFP-neo clones. (h) Dot plot cytograms show enrichment of EGFP-positive cells in Sox9-3′ EGFP knock-in embryos (top panel) and Sox9-EGFP/EGFP null chimeras (bottom panel). Only cells from a P1 population showing high green fluorescence were sorted. (i) RT–PCR analysis of Sox9 expression using total RNA extracted from sorted EGFP-positive cells of Sox9-3′ EGFP knock-in embryos and Sox9-EGFP/EGFP null chimeras. Figure 1: Generation of Sox9-3′ EGFP knock-in mice and Sox9-EGFP/EGFP null chimeras. ( a ) The structure of the genomic Sox9 locus, targeting vector and targeted allele for Sox9-3′ EGFP knock-in mouse is indicated. Exons are depicted as closed boxes and intronic sequences are shown as solid lines. DNA fragments detected by Southern blot analysis are indicated by double arrows, with the restriction enzymes and the probe. The IRES-EGFP-pA/loxP-flanked PGK-neo-bpA cassette is depicted as open boxes. B, Bam HI; P, Pst 1; E, Eco RI; X, Xba I; Bg, Bgl II; H, Hpa I. ( b ) Southern blot analysis of genomic DNA. Genomic DNA isolated from ES cell clones was digested with Bgl II and was then hybridized with the 3′ probe. The wild-type and mutant alleles were detected as 3 kb and 6.5 kb fragments, respectively. ( c ) EGFP expression in E9.5, E13.5 and E16.5 Sox9-3′ EGFP knock-in embryos. EGFP expression was detectable in a Sox9-specific pattern during embryogenesis. Scale bars, 500 μm (E9.5); 2 mm (E13.5) and 3 mm (E16.5). ( d ) The structure of the genomic Sox9 locus, targeting vector and targeted allele for Sox9-EGFP/EGFP null chimera is indicated. DNA fragments detected by Southern blot analysis are indicated by double arrows. ( e ) Southern blot analysis of genomic DNA. Genomic DNA isolated from ES cell clones was digested with Eco RI and was then hybridized with the 3′ probe. Wild-type and mutant alleles were detected as 7.1 kb and 5.8 kb fragments, respectively. ( f ) Southern blot analysis of the neo-deleted Sox9 EGFP clones after Cre recombination. The neo-deleted Sox9 EGFP allele was detected as a 4.2 kb fragment. ( g ) Southern blot analysis of the neo-deleted Sox9 EGFP/EGFP-neo clones. ( h ) Dot plot cytograms show enrichment of EGFP-positive cells in Sox9-3′ EGFP knock-in embryos (top panel) and Sox9-EGFP/EGFP null chimeras (bottom panel). Only cells from a P1 population showing high green fluorescence were sorted. ( i ) RT–PCR analysis of Sox9 expression using total RNA extracted from sorted EGFP-positive cells of Sox9-3′ EGFP knock-in embryos and Sox9-EGFP/EGFP null chimeras. Full size image The purity of EGFP-positive cells of Sox9-3′ EGFP knock-in and Sox9-EGFP/EGFP null chimeric embryos harvested from limb buds at embryonic day 12.5 (E12.5) was 96.0 and 94.8%, respectively ( Fig. 1h ), and reverse transcription (RT)–PCR analysis revealed that the expression of Sox9 in the majority of the population of cells isolated from Sox9-EGFP/EGFP null chimeras was deleted ( Fig. 1i ). Following the first screening of the microarray analysis (the complete annotated data set is available from the ArrayExpress repository, accession number E-MTAB-537), we further narrowed down the Sox9-related candidate genes using in situ hybridization in limb buds of E12.5 wild-type and conditional Sox9 knockout embryos harbouring the Prx1-Cre transgene. With the exception of Sox5 , Sox6 , Col2a1 , Col9a1 , Col9a3 and Col11a1 , 27 genes that exhibited the same pattern as Sox9 in conditional Sox9 knockout embryos were identified as Sox9-related genes involved in chondrogenesis ( Supplementary Table S1 ). Wwp2 showed 6.24-fold change in mRNA expression. Wwp2 is a downstream target of Sox9 The mRNA of Wwp2 is expressed in various adult mouse tissues, whereas Sox9 mRNA is detected in specific tissues ( Supplementary Fig. S1a,b ). During limb bud development in mouse embryos, Wwp2 was expressed during mesenchymal condensations of limb buds at E12.5, and then in periarticular and proliferating chondrocytes at E16.5 ( Fig. 2a ). These expression patterns of Wwp2 during chondrogenesis coincided with that of Sox9 . The expression of Wwp2 mRNA was completely abolished by the conditional inactivation of Sox9 using Prx1-Cre -mediated recombination in the limbs at E12.5 and Col2a1-Cre -mediated recombination in chondrocytes at E16.5 ( Fig. 2a ). Furthermore, adenoviral overexpression of Sox9 in ATDC5 cells, a clonal murine chondrogenic cell line, induced the upregulation of Wwp2 significantly ( Fig. 2b ); in contrast, knockdown of Sox9 using short interfering RNA (siRNA) led to significant downregulation of its expression ( Fig. 2b ), and the expression of Wwp2 protein also showed a Sox9 dependency ( Supplementary Fig. S1c,d ). Thus, these results indicate that Wwp2 is a downstream target of Sox9 , in vivo and in vitro . 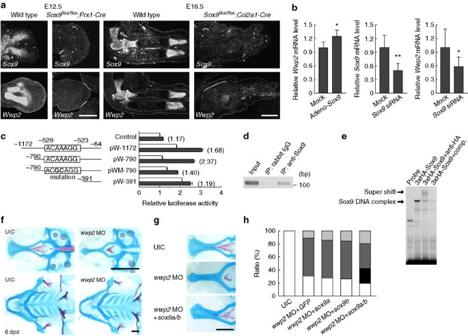Figure 2:Wwp2is identified as a downstream target of Sox9 and regulates palatogenesis. (a)In situhybridization ofSox9andWwp2in limb buds of wild-type,Sox9flox/floxPrx1-Cre(E12.5) andSox9flox/floxCol2a1-Cre(E16.5) mice. Scale bar, 500 μm. (b) Analysis ofWwp2mRNA expression levels by quantitative RT–PCR (qRT–PCR) in ATDC5 cells. ATDC5 cells were infected with human Sox9-expressing adenovirus (left panel) or transfected with 150 nM of siRNA for Sox9 (right panel; mean ± s.d.; *P<0.05; **P<0.01;n=5). (c) Luciferase promoter analysis using truncated forms of theWwp2promoter in the presence or absence of the Sox9 expression vector. HEK293 cells were transfected with the pW−1172(nt −1172 to −64), the pW−790(nt −790 to −64), the pW−391(nt −391 to −64) or the pWM−790plasmid, which includes a 2 bp substitution mutation, in the presence (black bars) or absence (white bars) of Sox9 expression vector. The value in brackets represents the Sox9-dependent increase in ratio (mean ± s.d.;n=4). (d) The specific binding of Sox9 to theWwp2promoter element detected by ChIP assay using ATDC5 cells. DNA–protein complex was immunoprecipitated by anti-Sox9 antibody. (e) EMSA revealed the specific binding of Sox9 to theWwp2promoter element. comp., competitor (unlabelled probe). (f) Small and fused palate in zebrafish carrying morpholino-mediated knockdown ofwwp2at 6 dpf. Zebrafish embryos were stained with alcian blue and alizarin red. UIC, uninjected control; MO, morpholino-treated animals. Scale bar, 200 μm. (g,h) RNA rescue experiments forwwp2knockdown in zebrafish usingsox9aand/orsox9b. (g) Palatal malformation induced bywwp2knockdown was partially rescued by the co-injection ofsox9aandsox9b. Scale bar, 100 μm. (h) Single injection ofsox9aorsox9bdid not rescue the palatal malformation induced bywwp2knockdown. UIC;n=51,wwp2MO+GFP;n=142,wwp2MO+sox9a;n=111,wwp2MO+sox9b;n=109,wwp2MO+sox9a/b;n=92 (white, normal; black, partial rescue; dark grey, fused and/or small; light grey, death). Figure 2: Wwp2 is identified as a downstream target of Sox9 and regulates palatogenesis. ( a ) In situ hybridization of Sox9 and Wwp2 in limb buds of wild-type, Sox9 flox/flox Prx1-Cre (E12.5) and Sox9 flox/flox Col2a1-Cre (E16.5) mice. Scale bar, 500 μm. ( b ) Analysis of Wwp2 mRNA expression levels by quantitative RT–PCR (qRT–PCR) in ATDC5 cells. ATDC5 cells were infected with human Sox9-expressing adenovirus (left panel) or transfected with 150 nM of siRNA for Sox9 (right panel; mean ± s.d. ; * P <0.05; ** P <0.01; n =5). ( c ) Luciferase promoter analysis using truncated forms of the Wwp2 promoter in the presence or absence of the Sox9 expression vector. HEK293 cells were transfected with the pW −1172 (nt −1172 to −64), the pW −790 (nt −790 to −64), the pW −391 (nt −391 to −64) or the pWM −790 plasmid, which includes a 2 bp substitution mutation, in the presence (black bars) or absence (white bars) of Sox9 expression vector. The value in brackets represents the Sox9-dependent increase in ratio (mean ± s.d. ; n =4). ( d ) The specific binding of Sox9 to the Wwp2 promoter element detected by ChIP assay using ATDC5 cells. DNA–protein complex was immunoprecipitated by anti-Sox9 antibody. ( e ) EMSA revealed the specific binding of Sox9 to the Wwp2 promoter element. comp., competitor (unlabelled probe). ( f ) Small and fused palate in zebrafish carrying morpholino-mediated knockdown of wwp2 at 6 dpf. Zebrafish embryos were stained with alcian blue and alizarin red. UIC, uninjected control; MO, morpholino-treated animals. Scale bar, 200 μm. ( g , h ) RNA rescue experiments for wwp2 knockdown in zebrafish using sox9a and/or sox9b . ( g ) Palatal malformation induced by wwp2 knockdown was partially rescued by the co-injection of sox9a and sox9b . Scale bar, 100 μm. ( h ) Single injection of sox9a or sox9b did not rescue the palatal malformation induced by wwp2 knockdown. UIC; n =51, wwp2 MO+ GFP ; n =142, wwp2 MO+ sox9a ; n =111, wwp2 MO+ sox9b ; n =109, wwp2 MO+ sox9a/b ; n =92 (white, normal; black, partial rescue; dark grey, fused and/or small; light grey, death). Full size image Wwp2 transcription is regulated directly by Sox9 Next, we assessed whether Sox9 regulates the transcription of Wwp2 directly. Putative Sox9-binding sites in the Wwp2 promoter region that are highly conserved among mammals (human, rat and mouse) were examined using in silico homology searches. A search of the region up to 4,000 nucleotides (nt) of Wwp2 exon 1 identified a putative Sox9-binding sequence (ACAAAGG), which lies between nt −529 and −523 and includes a nearly consensus motif for the Sox9-specific DNA-binding element [22] . To clarify the activity of the putative Sox9-responsive element of the Wwp2 promoter, a luciferase reporter assay was performed using a series of truncated fragments of the Wwp2 promoter cloned into a luciferase reporter vector ( Fig. 2c ). The results showed that co-transfection of pW −790 (which contains the Wwp2 promoter region from nt −790 to −64) and a Sox9 expression vector into HEK293 cells induced an approximately twofold increase in the relative reporter activity compared with that observed for the control ( Fig. 2c ). In addition, this increase in reporter activity was mostly abolished by using the mutated pW −790 (termed pWM −790 ) or pW −391 (which lacked the putative Sox9-binding motif). To obtain direct evidence of Sox9-mediated binding to this site, a chromatin immunoprecipitation (ChIP) assay was performed. The ChIP experiment using adenoviruses expressing Sox9 in ATDC5 cells detected the specific binding of Sox9 to the endogenous Wwp2 promoter element ( Fig. 2d ). Moreover, an electrophoretic mobility shift assay (EMSA) provided further evidence that HA-tagged Sox9 bound to the DNA fragment of this site ( Fig. 2e ). Hence, we conclude that Sox9 binds to the Wwp2 promoter element directly and transactivates Wwp2 expression. wwp2 knockdown induces palatal malformation in zebrafish In zebrafish, the expression of wwp2 in the cartilage of pharyngeal arches at 3 days post fertilization (dpf) was strongly reduced in embryos that were homozygous for sox9a or sox9b mutations ( Supplementary Fig. S2a ), whereas its expression in wild-type pharyngeal arches was detected at 2 dpf ( Supplementary Fig. S2b ). Interestingly, morpholino-mediated knockdown of wwp2 resulted in a small and fused palate, a phenotype that was reminiscent of sox9 -mutant zebrafish ( Fig. 2f ) [23] ; however, the expression of sox9a and sox9b , as detected in RT–PCR experiments, did not change after downregulation of wwp2 expression ( Supplementary Fig. S2c ). Furthermore, the co-injection of both sox9a and sox9b mRNA together with wwp2 morpholinos could partially rescue the palatal malformation ( Fig. 2g,h ). This restoration was thought to be due to the exogenous sox9-depedent induction of endogenous wwp2 expression. These findings would be expected under the hypothesis that Wwp2 has an essential role in chondrogenesis during palatogenesis, as an in vivo direct target of Sox9. Wwp2 interacts physically with Sox9 The similar palatal phenotype observed in sox9a -, sox9b - and wwp2 -deficient zebrafish raises the possibility of physical and functional interactions between Sox9 and Wwp2. An IP experiment of endogenous Sox9 and myc-tagged Wwp2 using ATDC5 cells showed that Sox9 physically interacted with Wwp2 ( Fig. 3a ). Co-IP experiments using deletion mutations of Sox9 ( Fig. 3b ) and Wwp2 ( Fig. 3c ) showed that the binding between Sox9 and Wwp2 was mediated by the carboxy terminal transactivation domain of Sox9 ( Fig. 3d ) and by the amino terminus (N-terminus) of Wwp2 ( Fig. 3e ), and not by the WW domains, which have a direct role in the mediation of specific and distinct interactions with Wwp2 substrates [24] . Indeed, Wwp2 did not stimulate ubiquitylation-mediated Sox9 degradation ( Supplementary Fig. S3 ). 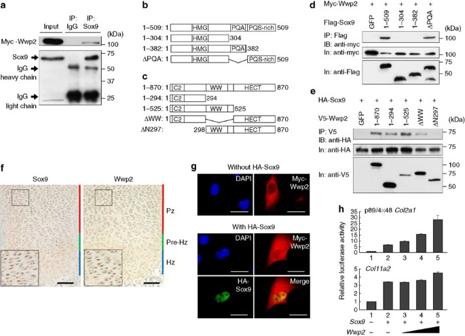Figure 3:Wwp2activates Sox9 by affecting its nuclear translocation. (a) Wwp2 interacted physically with endogenous Sox9 as demonstrated by IP assay using ATDC5 cells. Myc-taggedWwp2was transfected into ATDC5 cells and total cell lysates were immunoprecipitated 48 h after transfection using rabbit IgG (negative control) or an anti-Sox9 antibody, followed by immunoblotting with an anti-myc antibody. (b) Schematic images of Sox9 deletion mutations. Sox9 contains a high-mobility group domain (HMG, residues 104–182); a proline, glutamine and alanine domain (PQA, residues 339–379); and a proline, glutamine and serine-rich domain (PQS-rich, residues 402–509). (c) Schematic images of Wwp2 deletion mutations. Wwp2 contains a calcium-dependent membrane targeting domain (C2, residues 19–115), four tryptophan-based WW domains (WW, residues 300–477) and a carboxy terminus domain that is homologous to that of E6-AP (HECT, residues 525–870). (d) Co-immunoprecipitation assays between myc-tagged Wwp2 and Flag-tagged deletion mutations of Sox9. GFP expression plasmid was used as a negative control. IB, immunoblotting; In, input. (e) Co-immunoprecipitation assays between HA-tagged Sox9 and V5-tagged deletion mutations of Wwp2. GFP expression plasmid was used as a negative control. (f) Immunohistochemical analysis of Sox9 and Wwp2 in wild-type mouse limbs at E16.5 (DAB staining). Pz, proliferative zone; Pre-Hz, prehypertrophic zone; Hz, hypertrophic zone. Scale bar, 100 μm. (g) Nuclear translocation of Wwp2 in the presence or absence of exogenously overexpressed Sox9 in C3H10T1/2 cells. The nuclear translocation of Wwp2 was associated with Sox9. Scale bar, 20 μm. (h) Luciferase reporter assay using the p89/4×48Col2a1reporter plasmid orCol11a2reporter plasmid in C3H10T1/2 cells. The reporter activities increased in a Wwp2 dose-dependent manner (mean ± s.d.;n=5). Figure 3: Wwp2 activates Sox9 by affecting its nuclear translocation. ( a ) Wwp2 interacted physically with endogenous Sox9 as demonstrated by IP assay using ATDC5 cells. Myc-tagged Wwp2 was transfected into ATDC5 cells and total cell lysates were immunoprecipitated 48 h after transfection using rabbit IgG (negative control) or an anti-Sox9 antibody, followed by immunoblotting with an anti-myc antibody. ( b ) Schematic images of Sox9 deletion mutations. Sox9 contains a high-mobility group domain (HMG, residues 104–182); a proline, glutamine and alanine domain (PQA, residues 339–379); and a proline, glutamine and serine-rich domain (PQS-rich, residues 402–509). ( c ) Schematic images of Wwp2 deletion mutations. Wwp2 contains a calcium-dependent membrane targeting domain (C2, residues 19–115), four tryptophan-based WW domains (WW, residues 300–477) and a carboxy terminus domain that is homologous to that of E6-AP (HECT, residues 525–870). ( d ) Co-immunoprecipitation assays between myc-tagged Wwp2 and Flag-tagged deletion mutations of Sox9. GFP expression plasmid was used as a negative control. IB, immunoblotting; In, input. ( e ) Co-immunoprecipitation assays between HA-tagged Sox9 and V5-tagged deletion mutations of Wwp2. GFP expression plasmid was used as a negative control. ( f ) Immunohistochemical analysis of Sox9 and Wwp2 in wild-type mouse limbs at E16.5 (DAB staining). Pz, proliferative zone; Pre-Hz, prehypertrophic zone; Hz, hypertrophic zone. Scale bar, 100 μm. ( g ) Nuclear translocation of Wwp2 in the presence or absence of exogenously overexpressed Sox9 in C3H10T1/2 cells. The nuclear translocation of Wwp2 was associated with Sox9. Scale bar, 20 μm. ( h ) Luciferase reporter assay using the p89/4×48 Col2a1 reporter plasmid or Col11a2 reporter plasmid in C3H10T1/2 cells. The reporter activities increased in a Wwp2 dose-dependent manner (mean ± s.d. ; n =5). Full size image Wwp2 promotes the transcriptional activity of Sox9 To elucidate whether Wwp2 is associated with Sox9 transcriptional activity, we investigated the nuclear localization of Wwp2 in chondrocytes, the nuclear translocation of Wwp2 in the presence or absence of exogenously expressed Sox9, and then performed luciferase reporter assays using a chondrocyte-specific p89/4×48 Col2a1 reporter and a Col11a2 reporter construct. Immunohistochemical staining exhibited the abundant nuclear localization of Sox9 and Wwp2 in proliferating and pre-hypertrophic chondrocytes of mouse limb buds at E16.5 ( Fig. 3f ). Interestingly, in vitro multiple immunofluorescence (IF) of C3H10T1/2 cells, mouse pluripotent embryonic mesenchymal cell lines, co-transfected with HA-tagged Sox9 and/or myc-tagged Wwp2 revealed that the exogenously expressed Sox9 induced nuclear translocation of Wwp2 ( Fig. 3g and Supplementary Fig. S4 for lower magnification image). This result indicates that Sox9 mediates the recruitment of Wwp2 from the cytosol into the nucleus in chondrocytes. Furthermore, Wwp2 co-transfected with Sox9 into C3H10T1/2 cells enhanced the Col2a1 and Col11a2 reporter activities in a dose-dependent manner ( Fig. 3h ). Thus, these results strongly suggest that Wwp2 promotes the transcriptional activity of Sox9 as a cofactor in the nucleus of chondrocytes. Wwp2 binds to Med25 in chondrocytes To identify the mechanism underlying the Wwp2-mediated promotion of Sox9 transcriptional activity in chondrocytes, we sought other Wwp2-interacting proteins directly in chondrocytes using a yeast two-hybrid screening approach and identified Med25. Med25 exhibited strong physical interaction with Wwp2 in yeast ( Fig. 4a ). The mRNA of Med25 was expressed in various adult mouse tissues ( Supplementary Fig. S5), and Med25 was detected in mouse limb bud chondrocytes at E16.5 ( Fig. 4b ). Med25 was reported as a specific target of the VP16 transcriptional activator [25] , and was shown to enhance retinoic acid receptor/retinoid X receptor-mediated transcription in co-operation with CBP and mediators [26] . In addition, in human disease, homozygous mutation of MED25 is responsible for Charcot–Marie–Tooth syndrome type 2B [27] . However, the molecular functions of Med25 in chondrogenesis remain unknown. 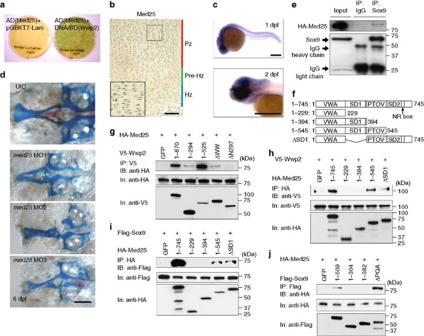Figure 4: Med25 is involved in palatogenesis and interacts physically with Sox9 and Wwp2. (a) Verification of the physical interaction between Wwp2 and Med25 by a yeast two-hybrid assay. The AH109 yeast strain was co-transformed with the pGADT7 vector expressing full-length Med25 and the pGBKT7-Lam vector (negative control; left dish), or the pGBKT7 vector expressing full-length Wwp2 (right dish) was cultured on SD/−Ade/−His/−Leu/−Trp/X-α-Gal high-stringency plates. (b) Immunohistochemical analysis of Med25 in a wild-type mouse limb at E16.5 (DAB staining). Scale bar, 100 μm. (c) Whole-mountin situhybridization ofmed25in zebrafish at 1 dpf (top panel) and 2 dpf (bottom panel). Scale bar, 500 μm. (d) Morpholino-mediated knockdown ofmed25in zebrafish induced palatal malformation. Three different kinds of palatal morphological malformations (med25MOs1–3) were observed. Scale bar, 100 μm. (e) Med25 interacted physically with endogenous Sox9 detected by IP assay using ATDC5 cells. HA-taggedMed25was transfected into ATDC5 cells and a total cell lysate was immunoprecipitated 48 h after transfection using rabbit IgG (negative control) or an anti-Sox9 antibody, followed by immunoblotting with an anti-HA antibody. (f) Schematic images of Med25 deletion mutations. Med25 contains a von Willebrand factor type A domain (VWA, residues 1–228), a synapsin I domain 1 (SD1, residues 229–381), a conserved region found in prostate tumour overexpressed protein 1 domain (PTOV, residues 395–545), an SD2 domain (residues 554–731) and an NR box (residues 646–650). (g–j) Co-immunoprecipitation assays using deletion mutations of Sox9, Wwp2 or Med25. GFP expression plasmid was used as a negative control. (g) Immunoprecipitation between HA-tagged full-length Med25 and V5-tagged deletion mutations of Wwp2. (h) Immunoprecipitation between V5-tagged full-length Wwp2 and HA-tagged deletion mutations of Med25. (i) Immunoprecipitation between Flag-tagged full-length Sox9 and HA-tagged deletion mutations of Med25. (j) Immunoprecipitation between HA-tagged full-length Med25 and Flag-tagged deletion mutations of Sox9. Figure 4: Med25 is involved in palatogenesis and interacts physically with Sox9 and Wwp2. ( a ) Verification of the physical interaction between Wwp2 and Med25 by a yeast two-hybrid assay. The AH109 yeast strain was co-transformed with the pGADT7 vector expressing full-length Med25 and the pGBKT7-Lam vector (negative control; left dish), or the pGBKT7 vector expressing full-length Wwp2 (right dish) was cultured on SD/−Ade/−His/−Leu/−Trp/X-α-Gal high-stringency plates. ( b ) Immunohistochemical analysis of Med25 in a wild-type mouse limb at E16.5 (DAB staining). Scale bar, 100 μm. ( c ) Whole-mount in situ hybridization of med25 in zebrafish at 1 dpf (top panel) and 2 dpf (bottom panel). Scale bar, 500 μm. ( d ) Morpholino-mediated knockdown of med25 in zebrafish induced palatal malformation. Three different kinds of palatal morphological malformations ( med25 MOs1–3) were observed. Scale bar, 100 μm. ( e ) Med25 interacted physically with endogenous Sox9 detected by IP assay using ATDC5 cells. HA-tagged Med25 was transfected into ATDC5 cells and a total cell lysate was immunoprecipitated 48 h after transfection using rabbit IgG (negative control) or an anti-Sox9 antibody, followed by immunoblotting with an anti-HA antibody. ( f ) Schematic images of Med25 deletion mutations. Med25 contains a von Willebrand factor type A domain (VWA, residues 1–228), a synapsin I domain 1 (SD1, residues 229–381), a conserved region found in prostate tumour overexpressed protein 1 domain (PTOV, residues 395–545), an SD2 domain (residues 554–731) and an NR box (residues 646–650). ( g – j ) Co-immunoprecipitation assays using deletion mutations of Sox9, Wwp2 or Med25. GFP expression plasmid was used as a negative control. ( g ) Immunoprecipitation between HA-tagged full-length Med25 and V5-tagged deletion mutations of Wwp2. ( h ) Immunoprecipitation between V5-tagged full-length Wwp2 and HA-tagged deletion mutations of Med25. ( i ) Immunoprecipitation between Flag-tagged full-length Sox9 and HA-tagged deletion mutations of Med25. ( j ) Immunoprecipitation between HA-tagged full-length Med25 and Flag-tagged deletion mutations of Sox9. Full size image med25 knockdown induces palatal malformation in zebrafish To clarify the role of Med25 in chondrogenesis, we investigated the in vivo functions of Med25 for skeletal formation in zebrafish. In situ hybridization showed that med25 was broadly expressed in the head, body and tail at 1 and 2 dpf ( Fig. 4c ). Intriguingly, morpholino-mediated knockdown of med25 in zebrafish resulted in palatal malformation ( Fig. 4d ), which closely resembled the palatal phenotype of wwp2 or sox9 mutants [23] ( Fig. 2f ). Furthermore, these palatal malformations could not be rescued by the co-injection of sox9a and sox9b mRNA or wwp2 mRNA ( Supplementary Fig. S6a,b ). Also, the injection of med25 mRNA with the wwp2 morpholinos had no influence on the palatal phenotype ( Supplementary Fig. S6c ). These findings suggest that Med25 transmits Sox9 transcriptional activity to general transcription machinery in association with Wwp2 in palatogenesis. Med25 interacts physically with Sox9 and Wwp2 The in vivo phenotypic similarities in palatogenesis between the knockdown of Sox9 , Wwp2 and Med25 , and the mutual interactions of Wwp2 with Sox9 and Med25, strongly suggest a functional communication between Sox9 and Med25 during chondrogenesis. Therefore, to assess whether Sox9 interacts physically and/or functionally with Med25, an IP assay was performed using ATDC5 cells transfected with HA-tagged Med25 . The result showed that Med25 interacted physically with endogenous Sox9 ( Fig. 4e ). Co-IP experiments using deletion mutations of Sox9 , Wwp2 and Med25 ( Figs 3b,c and 4f ) led to the following results. First, Med25 interacted physically with the N-terminus of Wwp2 and Wwp2 bound to the PTOV domain of Med25, which includes its transactivation domain [26] ( Fig. 4g,h ), and not to the SD1 domain of Med25, which contains the putative PY motif (the WW domains of Wwp2 have a preference for the PY motif in the binding of substrate proteins) [28] , [29] Indeed, Wwp2 did not stimulate ubiquitylation-mediated Med25 degradation ( Supplementary Fig. S7 ). Second, Med25 and Sox9 interacted with each transactivation domain ( Fig. 4i,j ). Thus, these physical interactions between Sox9, Wwp2 and Med25 suggest their functional interactions. In addition, multiple IF experiments revealed that Med25 was expressed in cell nucleus, and the nuclear translocation of Wwp2 depended on Sox9 and not on Med25 ( Supplementary Fig. S8a,b ). Wwp2 and Med25 augment Sox9 transcriptional activity Luciferase reporter assays using the p89/4×48 Col2a1 reporter or the Col11a2 reporter showed that co-transfection with Sox9 , Wwp2 and Med25 enhanced reporter activity significantly compared with that observed for Sox9 and Wwp2 or for Sox9 and Med25 ( Fig. 5a ). Interestingly, Wwp2 carrying a mutation in the HECT domain, which leads to loss of its catalytic function as an E3 ligase ( Wwp2-CA ; change of the cysteine residue at position 838 to an alanine), was still capable of increasing Sox9-dependent Col2a1 and Col11a2 luciferase activity ( Fig. 5a ). However, the slightly lower luciferase activity observed when using Wwp2-CA would indicate a loss of ubiquitylation-dependent activation by other molecules that regulate the transcription of Col2a1 and Col11a2 . Knockdown of either Wwp2 or Med25 in C3H10T1/2 cells resulted in significant downregulation of Col2a1 transcripts ( Fig. 5b,c ). In addition, this in vitro downregulation was not restored by adenoviral overexpression of Sox9 ( Fig. 5d ), which strongly suggests that Wwp2 and Med25 are key mediators of Sox9-dependent transcription. 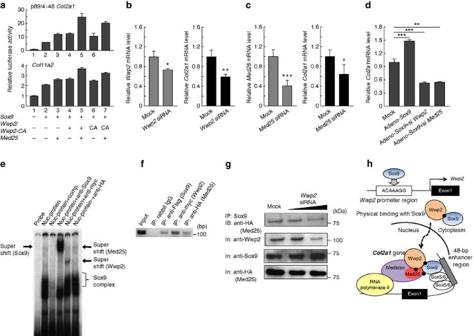Figure 5: Wwp2 mediates formation of transcriptional complex with Sox9 and Med25 and regulates Sox9 transcriptional activity. (a) Luciferase reporter assay using the p89/4×48Col2a1reporter andCol11a2reporter plasmid in C3H10T1/2 cells.Wwp2-CAincludes a mutation in the HECT domain ofWwp2. (mean ± s.d.;n=5). (b,c) Knockdown ofWwp2(b) orMed25(c) using siRNAs led to the downregulation ofCol2a1transcription in C3H10T1/2 cells detected by qRT–PCR. (mean ± s.d.; *P<0.05, **P<0.01, ***P<0.001;n=4). (d) Downregulation ofCol2a1induced by knockdown ofWwp2orMed25in C3H10T1/2 cells was not restored by exogenous Sox9 overexpression. (mean ± s.d.; Dunnett's test, **P<0.01; ***P<0.001;n=5). (e) EMSA using nuclear protein from C3H10T1/2 cells that were co-transfected with Flag-taggedSox9, myc-taggedWwp2and HA-taggedMed25. The 48-bpCol2a1enhancer oligonucleotide probe was used. Nuc-protein, nuclear protein. (f) ChIP assay detected recruitment of Sox9, Wwp2 and Med25 to the chondrocyte-specific enhancer region of theCol2a1gene. Cell lysate extracted from C3H10T1/2 cells that were co-transfected with Flag-taggedSox9, myc-taggedWwp2and HA-taggedMed25was immunoprecipitated with antibodies for each tag. (g) Downregulation of Wwp2 led to the attenuation of the physical binding between Sox9 and Med25. TheWwp2siRNA was initially transfected into ATDC5 cells and HA-taggedMed25was additionally transfected 24 h after transfection withWwp2siRNA. Nuclear protein was immunoprecipitated with an anti-Sox9 antibody, followed by immunoblotting with an anti-HA antibody. (h) Model describing the mechanism underlying the physical and functional interaction between Sox9, Wwp2 and Med25. Sox9 regulates the transcription ofWwp2and mediates the nuclear translocation of Wwp2, resulting in the formation of a transcriptional complex, including RNA polymerase II and Sox 5/6, which regulates the expression of theCol2a1gene. Figure 5: Wwp2 mediates formation of transcriptional complex with Sox9 and Med25 and regulates Sox9 transcriptional activity. ( a ) Luciferase reporter assay using the p89/4×48 Col2a1 reporter and Col11a2 reporter plasmid in C3H10T1/2 cells. Wwp2-CA includes a mutation in the HECT domain of Wwp2 . (mean ± s.d. ; n =5). ( b , c ) Knockdown of Wwp2 ( b ) or Med25 ( c ) using siRNAs led to the downregulation of Col2a1 transcription in C3H10T1/2 cells detected by qRT–PCR. (mean ± s.d. ; * P <0.05, ** P <0.01, *** P <0.001; n =4). ( d ) Downregulation of Col2a1 induced by knockdown of Wwp2 or Med25 in C3H10T1/2 cells was not restored by exogenous Sox9 overexpression. (mean ± s.d. ; Dunnett's test, ** P <0.01; *** P <0.001; n =5). ( e ) EMSA using nuclear protein from C3H10T1/2 cells that were co-transfected with Flag-tagged Sox9 , myc-tagged Wwp2 and HA-tagged Med25 . The 48-bp Col2a1 enhancer oligonucleotide probe was used. Nuc-protein, nuclear protein. ( f ) ChIP assay detected recruitment of Sox9, Wwp2 and Med25 to the chondrocyte-specific enhancer region of the Col2a1 gene. Cell lysate extracted from C3H10T1/2 cells that were co-transfected with Flag-tagged Sox9 , myc-tagged Wwp2 and HA-tagged Med25 was immunoprecipitated with antibodies for each tag. ( g ) Downregulation of Wwp2 led to the attenuation of the physical binding between Sox9 and Med25. The Wwp2 siRNA was initially transfected into ATDC5 cells and HA-tagged Med25 was additionally transfected 24 h after transfection with Wwp2 siRNA. Nuclear protein was immunoprecipitated with an anti-Sox9 antibody, followed by immunoblotting with an anti-HA antibody. ( h ) Model describing the mechanism underlying the physical and functional interaction between Sox9, Wwp2 and Med25. Sox9 regulates the transcription of Wwp2 and mediates the nuclear translocation of Wwp2, resulting in the formation of a transcriptional complex, including RNA polymerase II and Sox 5/6, which regulates the expression of the Col2a1 gene. Full size image Wwp2 forms a transcriptional complex with Sox9 and Med25 To obtain direct evidence of the formation of transcriptional complex through binding of these proteins to the chondrocyte-specific enhancer of the Col2a1 gene, we performed EMSA and ChIP assays using C3H10T1/2 cells, and revealed that Sox9, Wwp2 and Med25 were recruited onto the Col2a1 enhancer as a transcriptional complex ( Fig. 5e,f ). Importantly, knockdown of Wwp2 in ATDC5 cells attenuated the physical interaction between endogenous Sox9 and HA-tagged Med25 ( Fig. 5g ). Thus, these results indicate that Wwp2 mediates the interaction between Sox9 and Med25 via mutual physical binding and regulates Sox9 transcriptional activity. Here we identified Wwp2 as a Sox9 downstream target using FACS/microarray gene expression analysis and confirm the findings by in situ hybridization in conditional Sox9 knockout embryos and overexpression and knockdown of Sox9 in in vitro cells. Furthermore, both EMSA and ChIP assays using an anti-Sox9 antibody and reporter assays with luciferase reporter constructs indicate that Sox9 binds to the Wwp2 promoter and regulates Wwp2 expression directly. Zou et al . [30] recently reported that Wwp2 is detected in cartilaginous regions of the skull that are also positive for Sox9 and that Sox9 binds to an intronic region of Wwp2 , which mediates the Sox9-dependent expression of Wwp2 . Thus, these findings indicate that Sox9 regulates the cartilaginous expression of Wwp2 directly. Palatogenesis is controlled by multiple genetic factors, including genes encoding extracellular matrix proteins, growth factors and cell adhesion molecules. Alternations in the synthesis and accumulation of extracellular matrix proteins, including type II, IX, XI collagens, and proteoglycan [10] , [11] , [12] impair palatogenesis, all of that are regulated by Sox9 [1] , [7] , [8] , [9] . Indeed, mutations in or around SOX9 gene result in palatal malformations in human and a mouse model. Thus, it is obvious that Sox9 has a crucial role in palatogenesis. In this study, we show that Wwp2 is required for palatogenesis, mediated by formation of a transcriptional complex with Sox9 and Med25. Morpholino-mediated knockdown of wwp2 in zebrafish results in palatal malformation, which is comparable to that in Wwp2-deficient mice reported by Zou et al . [30] They also show that Wwp2 interacts with Goosecoid to facilitate its monoubiquitylation and augments its transcriptional activity for Sox6 expression [30] . Taking together with the previous findings that Sox6 cooperates with Sox9 to directly activate downstream target genes encoding extracellular matrix proteins [7] , [8] , it is likely that Wwp2 is essential for palatogenesis through Sox9 transcriptional activity (as shown in Fig. 5h ). Because Sox9 is required for the development of several tissues, which are characterized by very different genetic programs, other transcription factors and coactivators should provide specificity to the function of Sox9 in each of these cell types. Transcription factors form a large complex including the Mediator complex that conveys regulatory information from enhancer elements to the basal transcription machinery and acts as a bridge between transcription factors and RNA polymerase II. A recent study using human hepatocytes shows that Med25 is required for the recruitment of RNA polymerase II to the promoter of hepatocyte nuclear factor 4α and interacts with hepatocyte nuclear factor 4α through its transactivation domain [31] . Hence, it is likely that Med25 recruits RNA polymerase II on the promoter of Sox9 target genes. Med25 is believed to function in chromatin modification and pre-initiation complex assembly by recruiting CBP and the Mediator complex [26] . In addition, Trap230/Med12 is known as a coactivator of Sox9-dependent transcriptional regulation [14] . The phenotypic similarity in palatogenesis among sox9a / sox9b , wwp2 , med25 and Trap230 / med12 mutants [14] , [23] and the in vitro physical interaction between Sox9/Trap230, Sox9/Med25, Sox9/Wwp2 and Wwp2/Med25 may reflect a possible regulatory axis, which would include a Sox9–Wwp2–Med25–Trap complex. In conclusion, Sox9 stimulates Wwp2 expression and induces the translocation of Wwp2 into the nucleus of chondrocytes. Wwp2 mediates the binding between Sox9 and Med25, resulting in transactivation of target genes ( Fig. 5h ). This molecular mechanism is thought to be involved in palatogenesis in vivo . Our findings provide new insights into the regulatory mechanisms of Sox9 transcriptional activity during chondrogenesis and suggest new ideas regarding the molecular basis of the pathogenesis of cleft palate. Mice Sox9-3′ EGFP knock-in mice were generated using the targeting vector that spanned a 7.7 kb fragment of the mouse 129SvEv Sox9 gene [32] . An IRES-EGFP-pA/loxP-flanked PGK-neo-bpA cassette was inserted into an HpaI site within the 3′-untranslated region in exon 3. The targeting vector was introduced into PC3 mouse ES cells. Mouse chimeras were generated by injection of mutant ES cell clones into C57BL/6 host blastocysts; the resulting chimeras were bred with C57BL/6 mice to generate Sox9-3′ EGFP knock-in heterozygous mice. Sox9-EGFP/EGFP null chimeras were generated using a 4.5 kb NotI–SacII 5′ fragment and a 2.5 kb SacI–SacI 3′ fragment derived from the Sox9 locus [33] . An IRES-EGFP-pA/loxP-flanked PGK-neo-bpA cassette was introduced into the first exon of Sox9 , simultaneously deleting the translation start site and a portion of the high-mobility group DNA-binding domain. The targeting vector was introduced into AB-1 ES cells. To reuse G418 selection, the loxP-flanked neo cassette was excised from the Sox9 EGFP-neo/+ ES cell lines by transient expression of Cre recombinase. Neo-deleted Sox9 EGFP/+ ES cell clones were identified by Southern blot and verified by G418 selection. The Sox9 EGFP/+ ES cell lines were then retargeted with the original vector, as described above, and Sox9-EGFP/EGFP null ES cells were verified by Southern blot. The Sox9-EGFP/EGFP null ES cells were microinjected into C57BL/6 mouse blastocysts to generate chimeric embryos. Experimental procedures and animal maintenance followed institutional guidelines and were approved by local authorities. FACS and microarray analysis The limb buds of E12.5 Sox9-3′ EGFP knock-in and Sox9-EGFP/EGFP null chimeric embryos were dissected and dissociated into single cells using collagenase and disperse digestion. EGFP-positive cells were sorted using a FACSAria flow cytometer (Becton-Dickinson). Deletion of Sox9 in the cells harvested from Sox9-EGFP/EGFP null chimeric embryos was verified by PCR ( Supplementary Table S2 ). Total RNA was extracted and amplified according to the instructions provided by Affymetrix. Microarray analysis using the Affymetrix Mouse Genome 430 2.0 Array was performed according to the manufacturer's instructions. In situ hybridization of mouse embryos The development-associated expression patterns of Sox9 and Wwp2 mRNA in the limb buds of wild-type, Sox9 flox/flox Prx1-Cre and Sox9 flox/flox Col2a1-Cre embryos were analysed using the hybridization probes for Sox9 (255 bp) and Wwp2 (440 bp). Yeast two-hybrid screen A yeast two-hybrid assay was carried out using Matchmaker Library Construction & Screening Kits (Clontech), according to the manufacturer's instructions. The full-length mouse Wwp2 cDNA inserted into pGBKT7 was used as the bait vector. Med25 identified using a cDNA library from mouse rib chondrocytes was inserted into pGADT7 (prey vector). The pGADT7 vector expressing full-length Med25 was retransformed into the AH109 yeast strain, together with the pGBKT7 vector expressing Wwp2 or with the pGBKT7-Lam vector (negative control), and cultured on SD/−Ade/−His/−Leu/−Trp/X-α-Gal high-stringency plates. Zebrafish Developing and adult zebrafish were maintained using standard methods. Wild-type matings were obtained from the Oregon AB line. To suppress pigmentation, embryos were raised in zebrafish aquatic system water containing 1-phenyl-2-thiourea (0.003%) (Sigma). Zebrafish care was in accordance with the guidelines of the Children's Hospital Boston, University of Oregon and Murayama Medical Center. In situ hybridization of zebrafish Whole-mount in situ hybridization was carried out in zebrafish embryos at 1 and 2 dpf. Digoxigenin-labelled RNA probes were generated using the T7 and T3 labelling kit (Roche), according to the manufacturer's instructions. Signals were detected with an alkaline phosphatase-conjugated anti-digoxigenin antibody (Roche) and 4-nitro blue tetrazolium and 5-bromo-4-chloro-3-indolyl-phosphate. The primer sequences of the probes were described in Supplementary Table S2 . Morpholino knockdown and RNA rescue in zebrafish Gene Tools (Philomath; http://www.gene-tools.com ) supplied morpholino oligonucleotides (MOs) with the sequences: zebrafish wwp2 splice blocker-MO, 5′-CAGTGTGAATGCAGTGTTTTACCCA-3′ and zebrafish med25 ATG blocker, 5′-TATGGGTCACCTTTGGTCTACAGCC-3′. We injected one- or two-cell stage zebrafish embryos with ∼ 1–2 nl of morpholinos (20–25 ng for wwp2 splice blocker-MO and 5–10 ng for med25 ATG blocker). In RNA rescue experiments, we performed a series of experiments injecting each morpholino with either 50–500 pg of sox9a and/or sox9b , wwp2 or med25 mRNA. Zebrafish cartilage staining Zebrafish embryos at 4–7 dpf were stained with alcian blue and alizarin red and were flat mounted [34] . Images of stained, flat-mounted cartilages were captured using a Leica DMLB upright microscope and Spot camera (Diagnostic Instruments, Inc). siRNA The mouse Sox9 -specific siRNA (MISSION siRNA) was purchased from Sigma-Aldrich and the mouse Wwp2 - and Med25 -specific siRNAs (ON-TARGET plus SMARTpool) were purchased from Thermo Scientific Dharmacon. For mRNA expression analysis, each siRNA construct was transfected individually into ATDC5 or C3H10T1/2 cells (final concentration 150 nM) according to the manufacturer's protocol. Total RNA was extracted 48 h after transfection. A total of 1 μg of total RNA was used to synthesize cDNA using the Transcriptor First-Strand cDNA Synthesis Kit (Roche). Quantitative RT–PCR was performed using a LightCycler Instrument and a LightCycler FastStart DNA Master SYBR Green 1 Kit (Roche). The primer sequences for quantitative RT–PCR were described in Supplementary Table S2 . Luciferase assays In promoter analysis, mouse Wwp2 promoter fragments located upstream of the 5′-flanking region of exon 1 (−1,172 bp to −64 bp, −790 bp to −64 bp, and −391 bp to −64 bp) were subcloned into the pGL3-basic vector (Promega) to generate the Wwp2 promoter/luciferase reporter constructs, designated pW −1172 , pW −790 and pW −391 , respectively. The mutated pW −790 (termed pWM −790 ) construct, which includes a 2 bp substitution mutation in the nearly consensus binding site for high-mobility group box proteins, was produced using the QuickChange site-directed mutagenesis kit (Stratagene), according to the manufacturer's protocol. In Col2a1 or Col11a2 reporter analysis, a chondrocyte-specific p89/4×48 Col2a1 reporter or a Col11a2-luc reporter construct was used. pcDNA-renilla luciferase was used as an internal control. The plasmids were transfected using the FuGene HD transfection reagent (Roche) into HEK293 or C3H10T1/2 cells. Luciferase activity was assayed 48 h after transfection, according to the manufacturer's instructions. ChIP ChIP assays were performed using the ChIP Kit (Abcam), according to the manufacturer's protocol. ATDC5 cells cultured in six-well plates were infected with adenoviruses expressing Sox9; 48 h after infection, the fragments of cross-linked chromatin were immunoprecipitated with 3 μg of rabbit IgG (Cell signaling, 1 mg ml −1 ) or anti-Sox9 antibody (Chemicon, 1 mg ml −1 ). PCR primers were designed to contain a putative binding site within the mouse Wwp2 promoter region ( Supplementary Table S2 ). C3H10T1/2 cells were co-transfected with Flag-tagged Sox9, 6× myc-tagged Wwp2 and 3× HA-tagged Med25 expression vectors, and ChIP assay was performed according to the same scheme using 3 μg of anti-Flag (Abcam, 1 mg ml −1 ), anti-myc (Abcam, 1 mg ml −1 ) and anti-HA (Santa Cruz, 1 mg ml −1 ) antibodies. PCR was performed to detect the co-precipitation of the Col2a1 enhancer region ( Supplementary Table S2 ). EMSA A DNA probe corresponding to the putative Sox9 binding sequence of the 5′-flanking region of the Wwp2 gene was prepared by annealing complementary oligonucleotides ( Supplementary Table S2 ). The Sox9 protein was synthesized in vitro using a transcription/translation system (Promega). DNA-binding reactions and EMSA with the 48 bp Col2a1 enhancer probe were performed using nuclear proteins of C3H10T1/2 cells co-transfected with 6× myc-tagged Wwp2 and 3× HA-tagged Med25 expression vectors [35] ( Supplementary Table S2 ). Immunoprecipitation Tagged plasmids were transfected into ATDC5, C3H10T1/2 or HEK293 cells, and after 48 h, cells were lysed in buffer (50 mM Tris, 150 mM NaCl, 1 mM EDTA and 1% Triton X-100). Protein complexes were immunoprecipitated using protein G agarose with 3 μg of anti-Sox9 antibody (Chemicon, 1 mg ml −1 ), 3 μg of anti-V5 antibody (MBL, 1 mg ml −1 ), 30 μl of Ezview Red ANTI-FLAG M2 Affinity Gel (Sigma) or 30 μl of Anti-HA Affinity Matrix (Roche). Immunoprecipitated proteins were analysed by immunoblotting using each antibody. Immunohistochemical analysis Mouse limb buds at E16.5 were fixed in 4% paraformaldehyde and embedded in paraffin. Immunohistochemical analysis was performed using 3,3′-diaminobenzidine (DAB) staining (Zymed), and hematoxylin was used as a counterstain. The following primary antibodies were used: goat polyclonal anti-Sox9 antibody (Santa Cruz, 0.2 mg ml −1 ), rabbit polyclonal anti-AIP2 antibody (Santa Cruz, 0.2 mg ml −1 ) and goat polyclonal anti-Med25 antibody (Santa Cruz, 0.2 mg ml −1 ) diluted in antibody diluent (Zymed) to 1:100. IF staining IF staining was performed using C3H10T1/2 cells. Cells were fixed and permeabilized with cold methanol for 25 min at 4 °C. After washing, cells were blocked with a fresh blocking solution (4% donkey serum in PBS containing 0.05% Tween-20 (PBST)) for 30 min and were incubated with a rabbit anti-HA antibody (Santa Cruz, 0.2 mg ml −1 ) diluted to 1:200 in 1% donkey serum/PBS containing 0.05% Tween-20 for 1 h at room temperature. Cells were washed and incubated with an fluorescein isothiocyanate-conjugated donkey anti-rabbit IgG antibody (Jackson ImmunoResearch Laboratories, 0.5 mg ml −1 ), diluted to 1:1,000 for 1 h at room temperature. After washing, the procedure used for multiple staining was repeated using a goat anti-myc antibody (Abcam, 1 mg ml −1 ) or a goat anti-Flag antibody (Abcam, 1 mg ml −1 ; 1:200), and a TRITC-conjugated donkey anti-goat IgG antibody (1:1,000; Jackson ImmunoResearch Laboratories, 0.5 mg ml −1 ). Confocal images were obtained with a confocal laser microscope (Nikon Instruments Inc.). Statistical analysis Statistical evaluation was conducted using the Student's t -test or Dunnett's test. All error bars represent s.d. and significance was assessed as P <0.05. Accession codes: The microarray data have been deposited in ArrayExpress under the accession number E-MTAB-537. How to cite this article: Nakamura, Y. et al . Wwp2 is essential for palatogenesis mediated by the interaction between Sox9 and mediator subunit 25. Nat. Commun. 2:251 doi: 10.1038/ncomms1242 (2011).